gp96 expression in neutrophils is critical for the onset ofEscherichia coliK1 (RS218) meningitis Despite the fundamental function of neutrophils (polymorphonuclear leukocytes (PMNs)) in innate immunity, their role in Escherichia coli K1 (EC-K1) -induced meningitis is unexplored. Here we show that PMN-depleted mice are resistant to EC-K1 (RS218) meningitis. EC-K1 survives and multiplies in PMNs for which outer membrane protein A (OmpA) expression is essential. EC-K1 infection of PMNs increases the cell surface expression of gp96, which acts as a receptor for bacterial entry. Suppression of gp96 expression in newborn mice prevents the onset of EC-K1 meningitis. Infection of PMNs with EC-K1 suppresses oxidative burst by downregulating rac1, rac2 and gp91 phox transcription both in vitro and in vivo . The interaction of loop 2 of OmpA with gp96 is essential for EC-K1-mediated inhibition of oxidative burst. These results reveal that EC-K1 exploits surface-expressed gp96 in PMNs to prevent oxidative burst for the onset of neonatal meningitis. Bacterial meningitis remains a serious disease resulting in high morbidity and mortality, despite the use of potent antibiotics [1] , [2] , [3] . This unfavourable outcome is due to our incomplete knowledge about the pathogenesis of the disease for developing new modes of prevention. Escherichia coli K1 (EC-K1) is one of the most common pathogens causing neonatal meningitis [4] . The disease is fatal in 5–40% of infected neonates and causes neurological sequelae in up to 30% of survivors [5] . Studies in experimental models of haematogenous meningitis have shown that a certain threshold of bacteremia is necessary for the development of meningitis [6] , [7] . Thus, EC-K1 must avoid host defense mechanisms for proliferation in blood and/or tissues to reach a high level of bacteremia. Intracellular survival of EC-K1, therefore, represents a fundamental pathogenicity mechanism during the onset of meningitis. Several virulence factors have been implicated in the ability of EC-K1 (RS218) to cause meningitis, which include S-fimbria, IbeA, IbeB, cytotoxic necrotizing factor (CNF), TraJ and outer membrane protein A (OmpA) [8] , [9] , [10] , [11] , [12] , [13] . OmpA is one of the major outer membrane proteins of EC-K1 and has crucial roles in maintaining the integrity of outer membrane and in bacterial conjugation [14] , [15] , [16] . However, our studies demonstrate that OmpA is important for binding of EC-K1 to human brain microvascular endothelial cells (HBMEC) and subsequent invasion [10] . OmpA expression has also shown to be essential for survival of EC-K1 in immune cells such as macrophages and dendritic cells as well as to resist serum bactericidal activity [17] , [18] , [19] . We have subsequently shown that mutation of three residues in loops 1 and 2 prevent the interaction of EC-K1 with HBMEC and neutrophils [20] . Nonetheless, the role of neutrophils and how their interaction with EC-K1 OmpA contributes to the pathogenesis of EC-K1 meningitis is not well explored. Binding of microorganisms to polymorphonuclear leukocytes (PMN) surface-receptors generates signals that regulate the response of the phagocyte and killing of the microbial intruder [21] , [22] , [23] . Killing may be achieved through production of reactive oxygen species (ROS) at the expense of cytosolic nicotinamide adenine dinucleotide phosphate-oxidase (NADPH) [24] , [25] . However, pathogenic microbes develop strategies to avoid PMN killing by suppressing ROS generation [26] . Several studies have indicated that heat shock proteins such as gp96 can chaperone antigenic peptides and promote their delivery to antigen-presenting cells for presentation to T cells [27] . gp96 is an endoplasmic paralogue of heat shock protein 90 and has been shown to have a variety of roles in mammalian organisms [28] , [29] , [30] . Although gp96 is generally localized to the endoplasmic reticulum, it may gain extracellular access after cell activation, infection or necrotic cell death [31] , [32] , [33] . Our previous studies have shown that Ecgp96 (a homologue of gp96) acts as a receptor for OmpA of EC-K1 on HBMECs [10] . Therefore, we sought to investigate whether the interaction of EC-K1 with PMNs requires gp96. We observed that EC-K1 enters and survives in PMNs using gp96 as a receptor and suppresses the oxidative burst of PMNs for which OmpA expression is required. Interestingly, PMN-depleted or gp96 suppressed mice were resistant to EC-K1 meningitis, indicating that bacteria utilize PMNs as a replication permissive niche during initial stages of infection. PMN depletion in newborn mice prevents EC-K1 meningitis To determine whether neutrophils have a crucial role in the pathogenesis of EC-K1 meningitis, newborn mice were depleted of PMNs by injecting mAb RB6-8C5 starting at Day 1 and then infected intranasally with EC-K1 at Day 3. Flow cytometry analysis of spleen cells revealed complete depletion of PMNs in RB6-8C5-injected animals compared with wild-type (WT) or control-antibody (C-Ab)-injected mice ( Fig. 1a ). Unexpectedly, PMN-depleted mice survived without any visual signs of distress despite infection with EC-K1 beyond 7 days, whereas WT- and C-Ab-treated mice succumbed to infection by 96 h post-infection ( Fig. 1b ). PMN-depleted mice showed enhanced survival even at higher doses of EC-K1 ( Supplementary Fig. S1a and b ). A small number of bacteria that entered were cleared from circulation to undetectable levels by 48 h post-infection in PMN-depleted mice, whereas WT- and C-Ab-treated animals showed high degree of bacteremia ( Fig. 1c ). Cerebrospinal fluids (CSF) cultures were negative in PMN-depleted animals, indicating the absence of meningitis ( Fig. 1d ). The levels of proinflammatory cytokines, TNF-α, IL-1β, IL-6 and IL-12 were significantly higher in WT- and C Ab-treated infected mice compared with the levels in PMN-depleted mice ( Supplementary Fig. S1c–f ). Neither blood-brain barrier leakage nor bacterial load in the brains was observed in PMN-depleted mice ( Fig. 1e,f ). Histopathological examination of brain sections exhibited severe gliosis and increased cellularity in the molecular layer of the cortex in WT- and C-Ab-treated mice ( Fig. 1g ). Marked apoptosis indicated by pkynotic nuclei (inset), and infiltration of neutrophils was also observed in dentate gyrus in the hippocampus, whereas leptomeninges showed severe inflammation. In contrast, the brains from PMN-depleted mice showed no such pathological conditions. 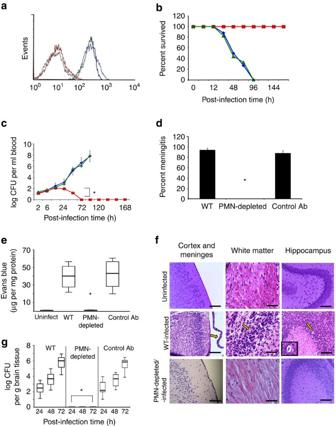Figure 1: PMN depletion renders newborn mice resistant toE. coliK1 meningitis. Newborn mice were injected four doses of mAb RB6-8C5 between day 1 and day 3 after birth or control antibody, and the depletion of PMNs in spleen was examined by flow cytometry. Isotype-matched antibody (grey line), WT (blue line), PMN-depleted (red line) or control antibody (green line) (a). WT (blue line), PMN-depleted (red line) or control antibody (green line) -treated mice at day 3 were infected withE. coliK1 and the percentage of survival was assessed (b). Bacteremia levels in these animals were determined by plating various dilutions of blood samples collected at indicated time points on agar containing antibiotics (c). CSF at 72 h post-infection were cultured in antibiotic containing Luria broth to assess the occurrence of meningitis (d). The blood-brain barrier permeability was determined by the Evans blue extravasation, as described in Methods section (e). Bacterial load in the brains of WT, PMN-depleted and control antibody-treated mice was evaluated after 72 h post-infection (f). Brains from WT- and PMN-depleted mice infected withE. coliK1 were removed and subjected to histopathological examination after staining with H and E (g). The data represent mean values ± s.d. and is representative of 5 independent experiments with 18 animals in each group. *P<0.01 PMN-depleted versus WT or control-Ab-treated mice by two-tailedt-test and ANOVA. Arrows indicate neutrophil infiltration in leptomeninges or white matter and apoptosis of neurons in hippocampus. Scale bars 20 μM. Figure 1: PMN depletion renders newborn mice resistant to E. coli K1 meningitis. Newborn mice were injected four doses of mAb RB6-8C5 between day 1 and day 3 after birth or control antibody, and the depletion of PMNs in spleen was examined by flow cytometry. Isotype-matched antibody (grey line), WT (blue line), PMN-depleted (red line) or control antibody (green line) ( a ). WT (blue line), PMN-depleted (red line) or control antibody (green line) -treated mice at day 3 were infected with E. coli K1 and the percentage of survival was assessed ( b ). Bacteremia levels in these animals were determined by plating various dilutions of blood samples collected at indicated time points on agar containing antibiotics ( c ). CSF at 72 h post-infection were cultured in antibiotic containing Luria broth to assess the occurrence of meningitis ( d ). The blood-brain barrier permeability was determined by the Evans blue extravasation, as described in Methods section ( e ). Bacterial load in the brains of WT, PMN-depleted and control antibody-treated mice was evaluated after 72 h post-infection ( f ). Brains from WT- and PMN-depleted mice infected with E. coli K1 were removed and subjected to histopathological examination after staining with H and E ( g ). The data represent mean values ± s.d. and is representative of 5 independent experiments with 18 animals in each group. * P <0.01 PMN-depleted versus WT or control-Ab-treated mice by two-tailed t -test and ANOVA. Arrows indicate neutrophil infiltration in leptomeninges or white matter and apoptosis of neurons in hippocampus. Scale bars 20 μM. Full size image Our observation that EC-K1 manipulates the function of macrophages for survival and cause meningitis [34] led us to hypothesize that PMNs provide initial safe havens for EC-K1 and subsequently hijack macrophages for their survival due to short lifespan of PMNs. To test this, we depleted PMNs in mice infected with EC-K1, 24 h post-infection. Interestingly, we observed that depleting PMNs after infection (PI-PMN-depleted) failed to prevent the onset of meningitis by EC-K1 ( Fig. 2a ). No statistical difference in blood bacterial load of PI-PMN-depleted, C-Ab-treated or WT mice was observed, and 90% of mice in all groups had meningitis with high bacterial titers in the brains ( Fig. 2b–d ). To further confirm these findings, PMNs and macrophages were isolated from WT-infected mice at 6- and 24 h post-infection, and intracellular bacteria enumerated. PMNs isolated at 6 h post-infection, not at 24 h post-infection, showed significantly greater number of bacteria inside the cells ( Fig. 2e ). In contrast, no bacteria were recovered from macrophages at 6 h, but only at 24 h post-infection. These results suggest that PMNs provide initial niche for EC-K1 and owing to short life span of PMNs, the bacteria subsequently take refuge in macrophages to survive and multiply. 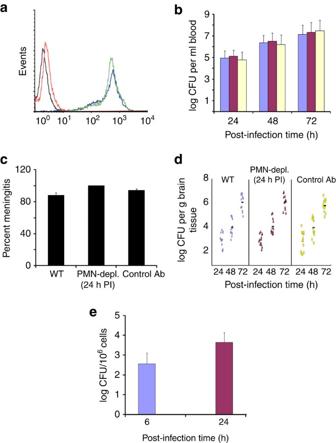Figure 2: PMN-depletion in mice after infection withE. coliK1 fails to prevent the onset of meningitis. Mice were infected withE. coliK1 (E44) and PMNs were depleted 24 h post-infection, as described in Methods section. The depletion of PMNs was confirmed by flow cytometry. Isotype-matched antibody (grey line), WT (blue line), PMN-depleted (red line) or control antibody (green line) (a). Blood from WT (blue bar), PMN-depleted (red bar) or control antibody-treated (yellow bar) mice was plated on antibiotic containing agar to determine bacteremia levels (b), CSF (c) and brain samples from WT (blue), PMN-depleted (red) or control antibody-treated (yellow) animals (d) were analysed for the presence ofE. coliK1 by growing the bacteria in antibiotic containing broth or on agar. PMNs (blue bar) and macrophages (red bar) were isolated from lungs of infected mice at 6 and 24 h post-infection and number of intracellular bacteria enumerated by plating on agar containing antibiotics (e). The data represent mean values ±s.d. and is representative of five independent experiments with 12 animals in each group. Figure 2: PMN-depletion in mice after infection with E. coli K1 fails to prevent the onset of meningitis. Mice were infected with E. coli K1 (E44) and PMNs were depleted 24 h post-infection, as described in Methods section. The depletion of PMNs was confirmed by flow cytometry. Isotype-matched antibody (grey line), WT (blue line), PMN-depleted (red line) or control antibody (green line) ( a ). Blood from WT (blue bar), PMN-depleted (red bar) or control antibody-treated (yellow bar) mice was plated on antibiotic containing agar to determine bacteremia levels ( b ), CSF ( c ) and brain samples from WT (blue), PMN-depleted (red) or control antibody-treated (yellow) animals ( d ) were analysed for the presence of E. coli K1 by growing the bacteria in antibiotic containing broth or on agar. PMNs (blue bar) and macrophages (red bar) were isolated from lungs of infected mice at 6 and 24 h post-infection and number of intracellular bacteria enumerated by plating on agar containing antibiotics ( e ). The data represent mean values ±s.d. and is representative of five independent experiments with 12 animals in each group. Full size image EC-K1 suppresses oxidative burst in PMNs for survival To examine whether EC-K1 survives inside PMNs, OmpA + E. coli (E44) and OmpA − E. coli (E91) were incubated with PMNs at an MOI of 10 for varying times. Although both bacteria entered PMNs efficiently, only OmpA + E. coli survived in PMNs, whereas OmpA − E. coli were killed within 2 h post-infection ( Fig. 3a,b ). To confirm whether OmpA expression is critical for survival in PMNs, OmpA − E. coli (E91) transfected with OmpA plasmid (pOmpA + ) or null plasmid (pOmpA − ) were used for phagocytosis assays. pOmpA + E. coli survived in PMNs, whereas pOmpA − E. coli were killed, indicating that OmpA expression is crucial for the survival ( Fig. 3a,b ). Furthermore, EC-K1 mutants that lack S-fimbria (Δsfa), IbeA (ΔibeA), type-1 fimbria (ΔfimH) or CNF (Δcnf) were used to examine the role of these virulence factors for survival in PMNs. All the mutants expressing OmpA were able to enter, survive and persist in PMNs similar to OmpA + E. coli ( Fig. 3c,d ). These findings confirm that other virulence factors, except OmpA, contribute insignificantly for the survival of EC-K1 in PMNs. To examine whether the survival of EC-K1 in PMNs was due to the suppression of ROS production, we monitored the ability of primary human PMNs to generate ROS following infection with EC-K1. Unstimulated PMNs did not produce detectable ROS, whereas PMNs treated with phorbol myristate acetate (PMA) potently generated ROS within 10 min ( Fig. 3e ). OmpA + E. coli failed to induce ROS production whereas a strong oxidative burst was documented in OmpA − E. coli -infected PMNs. ROS production in response to OmpA − E. coli was first detected after 5 min and reached a maximum between 40–45 min. Similar increase in oxidative burst was also observed with pOmpA − E. coli but not when infected with pOmpA + E. coli, E. coli ΔibeA, E. coli Δcnf, E. coli Δsfa, or E. coli ΔfimH strains ( Fig. 3f ). These data suggest that OmpA expression in EC-K1 and its interaction with PMNs is critical to prevent the oxidative burst and for survival in the cells. 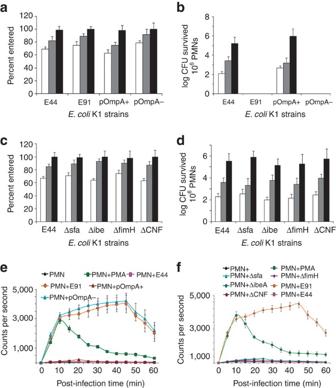Figure 3: Phagocytosis and oxidative burst inE. coliK1-infected PMNs. Various strains ofE. coliK1 were incubated with PMNs at a multiplicity of infection of 10 (PMN to bacteria ratio, 1:10) for indicated time points. The percentage uptake (a,c) and the number of intracellular bacteria (b,d) were determined by gentamicin protection assays at 2 h (white bar), 4 h (grey bar) and 6 h (black bar). In separate experiments, PMNs were left uninfected (PMN), stimulated with PMA, exposed to OmpA+E. coliK1 (E44), OmpA−E. coliK1 (E91),E. coliΔibeA,E. coliΔCNF,E. coliΔsfa,E. coliΔfimH or plasmid-complemented strains (pOmpA+and pOmpA−) ofE. coliK1, and the oxidative burst was measured using luminol-dependent chemiluminescence as described in Methods section (e, f). The data represent mean values ±s.d. of triplicate samples and is a representative of seven independent experiments. Figure 3: Phagocytosis and oxidative burst in E. coli K1-infected PMNs. Various strains of E. coli K1 were incubated with PMNs at a multiplicity of infection of 10 (PMN to bacteria ratio, 1:10) for indicated time points. The percentage uptake ( a , c ) and the number of intracellular bacteria ( b , d ) were determined by gentamicin protection assays at 2 h (white bar), 4 h (grey bar) and 6 h (black bar). In separate experiments, PMNs were left uninfected (PMN), stimulated with PMA, exposed to OmpA + E. coli K1 (E44), OmpA − E. coli K1 (E91), E. coli ΔibeA, E. coli ΔCNF, E. coli Δsfa, E. coli ΔfimH or plasmid-complemented strains (pOmpA + and pOmpA − ) of E. coli K1, and the oxidative burst was measured using luminol-dependent chemiluminescence as described in Methods section ( e, f ). The data represent mean values ±s.d. of triplicate samples and is a representative of seven independent experiments. Full size image Role of OmpA and effect of opsonization on ROS production To confirm the role of OmpA in preventing the production of ROS by PMNs, bacteria were pretreated with antibodies to OmpA before infecting PMNs. Anti-OmpA antibody pretreatment, or addition to the medium along with OmpA + E. coli (E44), led to a significant enhancement in the oxidative burst in PMNs, indicating that interaction of OmpA with PMNs is required for EC-K1-mediated suppressive effect on the oxidative burst capacity ( Fig. 4a ). Additionally, the effect of opsonization on oxidative burst was examined by pretreating the bacteria with pooled human serum, or heat-inactivated pooled human serum and then adding to PMNs. There was no increase in the ROS generation in PMNs infected with opsonized bacteria, which was similar to the untreated bacteria ( Fig. 4b ). This indicates that serum components may not have a significant role in the interaction of OmpA + E. coli with PMNs. Next, to determine whether viable EC-K1 interaction with PMNs is necessary for ROS generation, PMNs were infected with heat-killed (HK) OmpA + E. coli . Interestingly, HK-bacteria triggered strong ROS generation in PMNs that persisted for 60 min ( Fig. 4c ). However, when a mixture of viable and HK-bacteria in the ratio of 1:10 or 1:100 were added to PMNs, the PMN oxidative burst was completely prevented ( Fig. 4d ). We also observed that direct contact between PMN and bacteria is required because PMNs separated from OmpA + E. coli by 0.4-μm-pore transwells showed strong oxidative burst ( Supplementary Fig. S2a ). The reason for this oxidative burst may be due to the contribution of factors released by OmpA + E. coli , which passed through transwells and enhanced PMN ROS production. The bacterial culture supernatant from live OmpA + E. coli or bacterial lysates was found to be a potent stimulator of oxidative burst in PMNs ( Supplementary Fig. S2b ). OmpA + E. coli could suppress the ROS generation elicited by PMA or LPS before or after treatment of PMNs ( Fig. 4e ). OmpA + E. coli pretreated with chloramphenicol (Cm) elicited a strong oxidative burst in PMNs compared with untreated bacteria ( Fig. 4f ). However, a delay in adding Cm by 6 h, which allowed protein synthesis led to suppression of oxidative burst in OmpA + E. coli -infected PMNs. An increase in the ROS production was seen when tetracycline (tet), a cell-permeable antibiotic, was added to PMNs, thus preventing the multiplication of internal bacteria ( Fig. 4f ). These results suggest that live OmpA + E. coli that is capable of de novo protein synthesis actively inhibits the PMN respiratory burst. 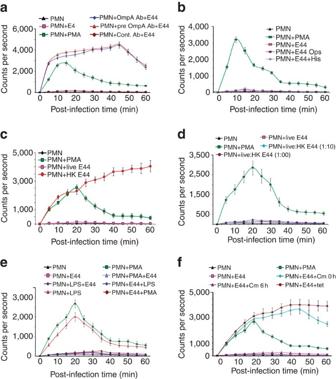Figure 4: Effect of anti-OmpA antibody and Cm on oxidative burst inE. coliK1-infected PMNs. PMNs were left uninfected, stimulated with PMA or infected with anti-OmpA antibody or control antibody-treatedE. coliK1. In these experiments, anti-OmpA antibodies were incubated withE. coliK1 before infection (PMN+pre OmpA Ab+E44) or added at the same time (PMN+OmpA Ab+E44) (a). PMNs were also infected withE. coliK1 unopsonized, opsonized with pooled human serum or treated with heat-inactivated serum (b). In separate experiments, PMNs were stimulated with HK bacteria alone (c) or a mixture of heat-killed and live bacteria (d). In addition, PMNs were first treated with PMA or LPS and then infected with OmpA+E. coliK1 (E44) or vice versa (e). Cm was added to PMN-bacteria co-culture immediately (PMN+E44+Cm 0 h) or after 6 h (PMN+E44+Cm 6 h) (f). Similarly, tetracycline (5 μg ml−1) was also added to PMN-bacteria co-culture (PMN+E44+tet). Oxidative burst was measured as described in Methods section after all these treatments. Data are expressed as mean values ±s.d. of triplicate samples and representative of five independent experiments. Figure 4: Effect of anti-OmpA antibody and Cm on oxidative burst in E. coli K1-infected PMNs. PMNs were left uninfected, stimulated with PMA or infected with anti-OmpA antibody or control antibody-treated E. coli K1. In these experiments, anti-OmpA antibodies were incubated with E. coli K1 before infection (PMN+pre OmpA Ab+E44) or added at the same time (PMN+OmpA Ab+E44) ( a ). PMNs were also infected with E. coli K1 unopsonized, opsonized with pooled human serum or treated with heat-inactivated serum ( b ). In separate experiments, PMNs were stimulated with HK bacteria alone ( c ) or a mixture of heat-killed and live bacteria ( d ). In addition, PMNs were first treated with PMA or LPS and then infected with OmpA + E. coli K1 (E44) or vice versa ( e ). Cm was added to PMN-bacteria co-culture immediately (PMN+E44+Cm 0 h) or after 6 h (PMN+E44+Cm 6 h) ( f ). Similarly, tetracycline (5 μg ml −1 ) was also added to PMN-bacteria co-culture (PMN+E44+tet). Oxidative burst was measured as described in Methods section after all these treatments. Data are expressed as mean values ±s.d. of triplicate samples and representative of five independent experiments. Full size image OmpA + E. coli reduces rac1, rac2 and gp91 phox transcription To assess whether EC-K1 had any effect on the expression of rac1 , rac2 and gp91 phox genes, encoding the multi-component NADPH oxidase complex responsible for oxidative burst in PMNs, RT–PCR was performed. A low level of rac1 transcript was detected in uninfected PMNs, which level was further dropped in OmpA + E. coli -infected cells, whereas OmpA − E. coli infection or PMA treatment enhanced the transcription levels ( Fig. 5a ). OmpA − E. coli and PMA stimulated PMNs exhibited a significant increase in rac2 and gp91 phox messenger RNA levels, whereas only low levels of transcripts was observed in OmpA + E. coli -infected cells. Quantitative analysis of PCR products normalized to gapdh levels revealed 70, 90 and 50% decrease in the expression of rac1 , rac2 and gp91 phox , respectively. in OmpA + E. coli -infected PMNs when compared with untreated cells ( Fig. 5b ). In contrast, PMNs incubated with OmpA − E. coli or PMA showed twofold increase in the transcription of these genes compared with unstimulated PMNs. Downregulation of Rac1, Rac2 and gp91 phox at the protein levels was also demonstrated on OmpA + E. coli infection, and upregulation of these molecules in OmpA − E. coli -infected or PMA-stimulated PMNs ( Fig. 5c,d ). Similarly, PMNs obtained from the spleens of E. coli -infected mice showed decreased levels of rac1 , rac2 and gp91 phox as compared with PMNs from uninfected mice ( Fig. 4e,f ; Supplementary Fig. S2c,d ). Overall, these data suggest that EC-K1 inhibits oxidative burst in PMNs both in vitro and in vivo by downregulating the expression of Rac1, Rac2 and gp91 phox . 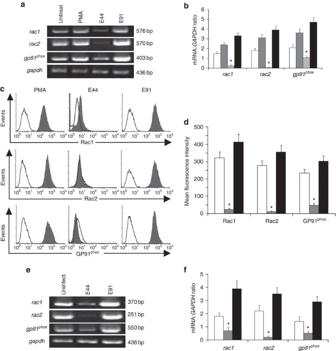Figure 5:E. coliK1 downregulates the transcription of NADPH oxidase components in PMNs. RT–PCR using primers forrac1,rac2 gp91phoxandgapdhand total RNA isolated from PMNs-untreated, PMA-stimulated, OmpA+E. coli(E44) -infected, or OmpA−E. coli(E91) -infected was performed (a). The densities of the transcripts from three different experiments were determined and mean values ±s.d. are expressed as a ratio ofrac1,rac2 gp91phoxmRNA andgapdhmRNA in untreated (white bar), PMA-treated (grey bar), E44-infected (shaded bar) or E91-infected (black bar) PMNs (b). In separate experiments, PMNs treated with PMA, OmpA+E. coli(E44) or OmpA−E. coli(E91) were washed, fixed, and the protein levels of Rac1, Rac2 and gp91phoxwere determined by flow cytometry using specific antibodies (c). For quantitative measurements, the geometric mean fluorescence intensities were plotted for Rac1, Rac2 and gp91phoxin PMA treated (white bar), E44-infected (grey bar) or E91-infected (black bar) PMNs (d). RT–PCR analysis of expression ofrac1,rac2 gp91phoxandgapdhmRNA in spleen PMNs isolated from uninfected, OmpA+E. coli(E44)-infected or OmpA−E. coli(E91) -infected mice (e). For quantitation, the transcription levels were determined by densitometry of bands from three different experiments and mean values ±s.d. are expressed as a ratio ofrac1,rac2 gp91phoxmRNA andgapdhin PMA treated (white bar), E44-infected (grey bar) or E91-infected (black bar) PMNs (f). The results presented in a–d are representative of seven independent experiments. *P<0.01 by two-tailedt-test and ANOVA. Figure 5: E. coli K1 downregulates the transcription of NADPH oxidase components in PMNs. RT–PCR using primers for rac1 , rac2 gp91 phox and gapdh and total RNA isolated from PMNs-untreated, PMA-stimulated, OmpA+ E. coli (E44) -infected, or OmpA − E. coli (E91) -infected was performed ( a ). The densities of the transcripts from three different experiments were determined and mean values ±s.d. are expressed as a ratio of rac1 , rac2 gp91 phox mRNA and gapdh mRNA in untreated (white bar), PMA-treated (grey bar), E44-infected (shaded bar) or E91-infected (black bar) PMNs ( b ). In separate experiments, PMNs treated with PMA, OmpA + E. coli (E44) or OmpA − E. coli (E91) were washed, fixed, and the protein levels of Rac1, Rac2 and gp91 phox were determined by flow cytometry using specific antibodies ( c ). For quantitative measurements, the geometric mean fluorescence intensities were plotted for Rac1, Rac2 and gp91 phox in PMA treated (white bar), E44-infected (grey bar) or E91-infected (black bar) PMNs ( d ). RT–PCR analysis of expression of rac1 , rac2 gp91 phox and gapdh mRNA in spleen PMNs isolated from uninfected, OmpA + E. coli (E44)-infected or OmpA − E. coli (E91) -infected mice ( e ). For quantitation, the transcription levels were determined by densitometry of bands from three different experiments and mean values ±s.d. are expressed as a ratio of rac1 , rac2 gp91 phox mRNA and gapdh in PMA treated (white bar), E44-infected (grey bar) or E91-infected (black bar) PMNs ( f ). The results presented in a–d are representative of seven independent experiments. * P <0.01 by two-tailed t -test and ANOVA. Full size image gp96 expression in PMNs is vital for EC-K1 entry We have demonstrated that Ecgp96 (HSP90β form) is a receptor for OmpA of EC-K1 in HBMEC [10] . Therefore, we theorize that gp96 on the surface of PMNs may be having a role in the infection. To test this, PMNs infected with EC-K1 were examined for the expression of gp96. OmpA + E. coli (E44) increased the expression of gp96 on PMNs on infection by sevenfold in comparison to uninfected cells ( Fig. 6a ). In contrast, the expression of gp96 in PMNs infected with OmpA − E. coli (E91) was similar to that of uninfected PMNs. Next, we determined whether gp96 has a role in the entry of EC-K1 in PMNs by suppressing the expression using short interfering RNA (siRNA). Although a majority of gp96 is confined to the cytosol, under certain conditions, some portions of gp96 translocate to plasma membrane [31] . Therefore, both extracellular and intracellular expression of gp96 was examined after the introduction of siRNAs. The expression of gp96 was considerably reduced in all siRNA-transfected PMNs while control-siRNA transfected cells showed no decrease in the expression ( Fig. 6b,c ). RT–PCR also revealed a drastic reduction in the transcript levels of gp96 in gp96-siRNA-1-transfected PMNs on infection with OmpA + E. coli ( Fig. 6d ). Of note, the entry of EC-K1 was inhibited by 80% in gp96-siRNA-1-transfected PMNs ( Fig. 6e ). Nonetheless, OmpA + E. coli that entered in low numbers were killed completely by 6 h post-infection in gp96-siRNA-1 transfected PMNs ( Fig. 6f ). As gp96 siRNA-1 significantly reduced the expression of gp96 in PMNs, this siRNA was used for subsequent experiments. No oxidative burst was observed in gp96 PMNs infected with EC-K1 owing to the lack of entry of a sufficient number of bacteria to mount ROS generation ( Fig. 5g ). Because knocking down gp96 can have an effect on other receptors, we blocked gp96 interaction with OmpA of EC-K1 by anti-gp96 antibodies. The entry, survival and the production of ROS were significantly reduced when PMNs were pretreated with anti-gp96 antibody ( Supplementary Fig. S3a-c ). These results suggest that EC-K1 utilizes gp96 on PMNs to enter and subsequently suppress the generation of oxidative burst. 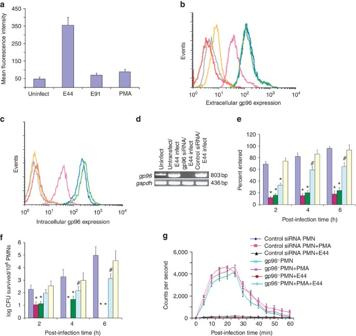Figure 6: The expression of gp96 in PMNs is critical forE. coliK1 entry and suppression of oxidative burst. PMNs were infected with OmpA+E. coli(E44), OmpA−E. coli(E91), stimulated with PMA or left without infection. The expression of gp96 on the surface of PMNs was determined by flow cytometry. The data are presented as geometric mean fluorescence intensity of logarithmic data subtracted from isotype-matched controls (a). In separate experiments, PMNs were transfected with three gp96 siRNAs (red line, orange line and pink line for gp96-siRNA-1, gp96-siRNA-2, gp96-siRNA-3, respectively) or control siRNA (green line), and the expression of extracellular (b) or intracellular (c) gp96 in PMNs was measured by flow cytometry. Isot-ype-matched control antibody (grey line) or untransfected PMNs (blue line) were used as controls. RT–PCR performed with gp96 specific primers and total RNA isolated from gp96-siRNA-1 or control siRNA-transfected PMNs or untransfected cells (d). The entry (e) and intracellular survival (f) of bacteria in PMNs transfected with gp96-siRNA-1 (red bar) or gp96-siRNA-2 (green bar) or gp96-siRNA-3 (blue bar) or control siRNA (yellow bar) or untransfected (purple bar) was determined. In addition, oxidative burst was also determined in gp96-siRNA-1-transfected PMNs and then treated with PMA, OmpA+E. coli(E44) or PMA+E44 (g). Data are expressed as the mean values ±s.d. of triplicate samples and are representative of five independent experiments. The oligo numbers for gp96-siRNA-1, gp96-siRNA-2, and gp96-siRNA-3 were HSS110955, HSS110953 and HSS186409, respectively. *P<0.01 or#P<0.05 by two-tailedt-test and ANOVA. Figure 6: The expression of gp96 in PMNs is critical for E. coli K1 entry and suppression of oxidative burst. PMNs were infected with OmpA + E. coli (E44), OmpA − E. coli (E91), stimulated with PMA or left without infection. The expression of gp96 on the surface of PMNs was determined by flow cytometry. The data are presented as geometric mean fluorescence intensity of logarithmic data subtracted from isotype-matched controls ( a ). In separate experiments, PMNs were transfected with three gp96 siRNAs (red line, orange line and pink line for gp96-siRNA-1, gp96-siRNA-2, gp96-siRNA-3, respectively) or control siRNA (green line), and the expression of extracellular ( b ) or intracellular ( c ) gp96 in PMNs was measured by flow cytometry. Isot-ype-matched control antibody (grey line) or untransfected PMNs (blue line) were used as controls. RT–PCR performed with gp96 specific primers and total RNA isolated from gp96-siRNA-1 or control siRNA-transfected PMNs or untransfected cells ( d ). The entry ( e ) and intracellular survival ( f ) of bacteria in PMNs transfected with gp96-siRNA-1 (red bar) or gp96-siRNA-2 (green bar) or gp96-siRNA-3 (blue bar) or control siRNA (yellow bar) or untransfected (purple bar) was determined. In addition, oxidative burst was also determined in gp96-siRNA-1-transfected PMNs and then treated with PMA, OmpA + E. coli (E44) or PMA+E44 ( g ). Data are expressed as the mean values ±s.d. of triplicate samples and are representative of five independent experiments. The oligo numbers for gp96-siRNA-1, gp96-siRNA-2, and gp96-siRNA-3 were HSS110955, HSS110953 and HSS186409, respectively. * P <0.01 or # P <0.05 by two-tailed t -test and ANOVA. Full size image Suppression of gp96 expression in vivo prevents meningitis If survival of EC-K1 inside PMNs represents a significant contribution to the pathogenesis of meningitis, then limiting access of the organism to this intracellular site should prevent the onset of meningitis. To test this, we suppressed the expression of gp96 in mice using gp96-siRNA-1 and Invivofectamine reagent [33] , [35] . No stimulation of immune response was detected with the administration of siRNA and Invivofectamine reagent as the cytokine levels (TNF-α, IL-1β, IL-6 and IL-12) were similar between treated and untreated mice ( Supplementary Fig. S4a–d ). Both extracellular and intracellular gp96 expression in PMNs obtained from spleen, peritoneum and liver was significantly suppressed in transfected mice, whereas control siRNA had no effect ( Fig. 7a ; Supplementary Fig. S5a ). RT–PCR confirmed knockdown of gp96 in PMNs in mice, even after infection with EC-K1 ( Supplementary Fig. S4b ). gp96 knockdown (KD) mice showed better survival compared with WT or control siRNA-treated mice, which succumbed to infection by 96 h post-infection ( Fig. 7b ). No bacteremia or blood-brain barrier leakage was observed in gp96 KD mice, whereas blood bacterial numbers or Evans blue leakage increased with post-infection time in WT mice ( Fig. 7c,d ). CSF cultures were positive in 90 and 100% of WT and control siRNA treated animals, respectively, whereas all the CSF cultures were sterile in gp96 KD mice ( Fig. 7e ). No bacteria were recovered from the brains of gp96 KD mice and histopathological examination of brain tissues revealed no brain damage ( Fig. 6f ; Supplementary Fig. S5c ). Because lack of PMNs prevents the onset of meningitis in newborn mice, these data suggest that gp96 expression in PMNs may be critical for the onset of meningitis by EC-K1. 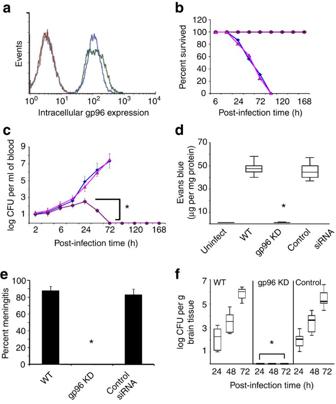Figure 7: Suppression of gp96 in newborn mice provides protection againstE. coliK1 meningitis. Newborn mice were injected with gp96-siRNA-1 to knockdown (KD) the expression of gp96, as described in Methods section and extracellular expression of gp96 in PMNs obtained from spleen of WT (blue line), gp96 KD (red line) or control siRNA-treated (green line) animals was assessed by flow cytometry (a). The grey line represents isotype-matched antibody control. WT (diamonds), gp96 KD (circles) or control siRNA-treated (triangles) mice at day 3 were infected withE. coliK1, and the survival of animals was recorded up to 7 days post-infection (b). Bacteremia levels in WT (diamonds), gp96-KD (circles) or control siRNA treated (triangles) and infected mice were determined at various times post-infection (c). In separate experiments, gp96 KD or WT mice infected withE. coliK1 were injected with Evans blue dye and leakage was determined as described in Methods sections (d). CSF samples (e) and brains (f) were collected and the presence of bacteria determined by culturing in antibiotic containing broth or on agar. The data represent mean values ±s.d. and is representative of five independent experiments with 18 animals in each group. *P<0.01 by two-tailedt-test, Fisher's exact test and ANOVA. Figure 7: Suppression of gp96 in newborn mice provides protection against E. coli K1 meningitis. Newborn mice were injected with gp96-siRNA-1 to knockdown (KD) the expression of gp96, as described in Methods section and extracellular expression of gp96 in PMNs obtained from spleen of WT (blue line), gp96 KD (red line) or control siRNA-treated (green line) animals was assessed by flow cytometry ( a ). The grey line represents isotype-matched antibody control. WT (diamonds), gp96 KD (circles) or control siRNA-treated (triangles) mice at day 3 were infected with E. coli K1, and the survival of animals was recorded up to 7 days post-infection ( b ). Bacteremia levels in WT (diamonds), gp96-KD (circles) or control siRNA treated (triangles) and infected mice were determined at various times post-infection ( c ). In separate experiments, gp96 KD or WT mice infected with E. coli K1 were injected with Evans blue dye and leakage was determined as described in Methods sections ( d ). CSF samples ( e ) and brains ( f ) were collected and the presence of bacteria determined by culturing in antibiotic containing broth or on agar. The data represent mean values ±s.d. and is representative of five independent experiments with 18 animals in each group. * P <0.01 by two-tailed t -test, Fisher's exact test and ANOVA. Full size image Loop 2 of OmpA interacts with gp96 in PMNs OmpA is a 325 amino-acid protein with 8 transmembrane domains and 4 extracellular loops [15] . 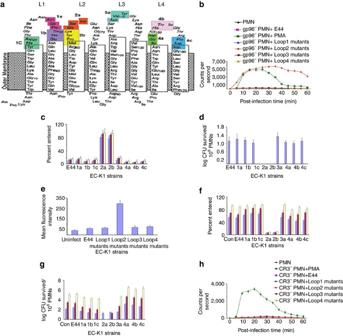Figure 8: Interaction of loop 2 of OmpA with gp96 in PMNs is necessary for the entry ofE. coliK1 and suppression of ROS production. VariousE. coliK1 (E44) mutants were generated by mutating three amino acids to alanines in the extracellular loops of OmpA (highlighted) (a). PMNs were transfected with gp96-siRNA-1 (gp96 PMNs) and oxidative burst capacity of PMNs infected withE. coliK1 mutants was examined (b). In addition, entry (c) and survival (d) ofE. coliK1 mutants was determined in gp96-siRNA-1-transfected PMNs at 2 h (purple bar), 4 h (maroon bar) and 6 h (yellow bar) post-infection. CR3 expression on the surface of PMNs infected withE. coliK1 mutants was analysed by flow cytometry. Mean fluorescence intensities were graphed (e). In separate experiments, PMNs were transfected with CR3 siRNA (CR3 PMNs) and the entry (f), survival (g) and oxidative burst capacity (h) of PMNs infected withE. coliK1 mutants was determined. Results are expressed as mean values ±s.d. of triplicate samples and are representative of five independent experiments. Therefore, next to determine which loops of OmpA interact with gp96 in PMNs, three to four amino acids of OmpA extracellular loops were mutated to alanines as shown in Figure 8a [20] . For convenient presentation of data, the loop mutants were divided into four groups. Mutations in loop 2 could not prevent the oxidative burst as compared with OmpA + E. coli (E44) or other loop mutants ( Fig. 8b ). To examine whether the interaction of gp96 with loop 2 domains in PMNs is necessary for EC-K1 entry, the expression of gp96 was suppressed using siRNA and then the cells infected with EC-K1. Loop 2 mutants (L2Ms) unexpectedly entered gp96 knockdown PMNs with a fourfold more frequency than other bacteria ( Fig. 8c ). However, L2Ms were killed in gp96 knockdown PMNs in a short time; whereas other loop mutants although entered in low numbers were killed by 4 h post-infection ( Fig. 8d ). As our previous studies revealed that CR3 expression in PMNs has a crucial role in killing of EC-K1, we speculated that L2Ms may have entered PMNs via CR3 and, subsequently, could not survive because of the oxidative burst [35] . Therefore, we examined the expression of CR3 on PMNs on infection with various OmpA loop mutants. L2Ms increased the expression of CR3, while other mutants showed CR3 expression similar to that of OmpA + E. coli ( Fig. 8e ). To confirm the role of CR3 in the entry of L2Ms, we suppressed the expression of CR3 in PMNs by siRNA, which reduced CR3 expression significantly ( Supplementary Fig. S6a ). Interestingly, L2Ms were unable to enter and survive in CR3 knockdown PMNs, whereas other mutants entered and survived ( Fig. 8f,g ). No oxidative burst was observed in CR3-knocked-down PMNs which were infected with L2Ms ( Fig. 8h ). Additionally, blocking of CR3 interaction with L2 M by a CR3-blocking peptide XVA143 prevented the entry of L2Ms into PMNs ( Supplementary Fig. S6b-h ), indicating that loop 2 regions dictate the interaction with either gp96 or CR3 depending on the peptide sequence. To confirm the role of CR3 and gp96, PMNs were transfected with gp96 and CR3 siRNA and then used for EC-K1 phagocytosis assays. None of the EC-K1 strains was able to enter and survive inside PMNs ( Supplementary Fig. S7a,b ). There was no oxidative burst observed in PMNs and could be due to the interaction of a low number of bacteria with the cells ( Supplementary Fig. S7c ). These results indicate that loop 2 of OmpA in EC-K1 interacts with gp96 on PMNs to enter, survive and prevent oxidative burst. Lack of this interaction enhances the expression of CR3 by which EC-K1 enters, however, could not survive in PMNs. Figure 8: Interaction of loop 2 of OmpA with gp96 in PMNs is necessary for the entry of E. coli K1 and suppression of ROS production. Various E. coli K1 (E44) mutants were generated by mutating three amino acids to alanines in the extracellular loops of OmpA (highlighted) ( a ). PMNs were transfected with gp96-siRNA-1 (gp96 PMNs) and oxidative burst capacity of PMNs infected with E. coli K1 mutants was examined ( b ). In addition, entry ( c ) and survival ( d ) of E. coli K1 mutants was determined in gp96-siRNA-1-transfected PMNs at 2 h (purple bar), 4 h (maroon bar) and 6 h (yellow bar) post-infection. CR3 expression on the surface of PMNs infected with E. coli K1 mutants was analysed by flow cytometry. Mean fluorescence intensities were graphed ( e ). In separate experiments, PMNs were transfected with CR3 siRNA (CR3 PMNs) and the entry ( f ), survival ( g ) and oxidative burst capacity ( h ) of PMNs infected with E. coli K1 mutants was determined. Results are expressed as mean values ±s.d. of triplicate samples and are representative of five independent experiments. Full size image Pathogenic bacteria have evolved efficient strategies to overcome the weaponry of neutrophils to win the combat [36] , [37] , [38] . An interesting observation in this study is that depletion of PMNs in newborn mice renders them resistant to EC-K1 infection. This indicates that interaction between PMN and EC-K1 interaction is a critical step in the pathogenesis of neonatal meningitis. As the bacterial numbers did not increase in PMN-depleted mice, PMNs may act as prime safe havens for the multiplication during initial stages of infection necessary to reach high-grade bacteremia. In addition, PMNs containing EC-K1 may disseminate bacteria to distal sites or to present to macrophages for a second round of multiplication. Concurrently, depletion of PMNs 24 h post-infection in mice could not protect them from the onset of meningitis. Another compelling observation is that OmpA + E. coli significantly upregulates the expression of gp96 in PMNs, which in turn acts as a receptor for OmpA for the entry of EC-K1 into the cells. Of note, silencing the expression of gp96 by siRNA in PMNs prevented the entry of EC-K1. Confirming the role of gp96 in EC-K1-induced pathogenesis, gp96 knockdown mice were resistant to EC-K1 meningitis, which is due to lack of high-grade bacteremia. The present study provides both in vitro and in vivo evidence that EC-K1 can exploit the inflammatory response of the host to facilitate its own survival by gaining access to a locale within PMN using gp96 where it is shielded from being killed. On contact with pathogens, PMNs undergo oxidative burst leading to the production of a large array of ROS [39] . NADPH oxidase system has a major role in the production of ROS [40] , [41] , [42] , [43] , [44] , [45] . As Rac1, Rac2 and gp91 phox have an essential role in the generation of oxidative burst in neutrophils, we examined the levels of these molecules in PMNs infected with EC-K1. Interestingly, we observed significant downregulation in the expression of Rac1, Rac2 and gp91 phox at both gene and protein levels. Although a number of pathogens has been demonstrated to modulate PMN oxidative metabolism, EC-K1 appears to utilize a unique mechanism to accomplish the downregulation of oxidative burst in PMNs. Helicobacter pylori and Salmonella enterica serovar typhimurium have been shown to stimulate the ROS generation in PMNs by redirecting NADPH oxidase activity away from the phagosome distinct than EC-K1, which prevents oxidative burst in PMNs by suppressing the expression of NADPH oxidase components [46] , [47] . Streptococcus pyogenes has been shown to trigger ROS generation in PMNs; however, this pathogen up-regulates oxidative stress response genes to avoid intracellular killing within PMN phagosomes [48] . Other bacteria such as Yersinia pestis , Yersinia pseudotuberculosis and Yersinia enterocolitica inhibit phagocytosis by PMNs employing a variety of effector proteins like YopT and YopO [26] . However, we observed that EC-K1-mediated suppression of oxidative burst in PMNs depends on OmpA as EC-K1 mutants that were defective in the expression of other virulence factors including FimH, CNF, S-fimbrial adhesin and ibeA failed to trigger the production of ROS. However, OmpA − E. coli triggered a strong oxidative burst in PMNs, indicating that OmpA, but not other virulence factors, have an important role in the ability of EC-K1 to downregulate oxidative burst in PMNs. Interestingly, EC-K1 also blocked PMA or LPS-induced oxidative burst in PMNs unlike Neisseria gonorrhoea that do not prevent PMA-mediated oxidative burst in PMNs [49] . Besides, this EC-K1-mediated suppressive effect on ROS generation requires live proliferating bacteria and a direct contact between bacteria and PMNs. Bacterial protein synthesis is required for EC-K1 to block the PMN oxidative burst because bacteriostatic concentrations of Cm prevent this effect induced by the bacterium. Nevertheless, bacterial lysates, killed bacteria and bacterial supernatants were able to induce strong ROS production in PMNs. This finding implies that PMNs have the ability to recognize and respond to EC-K1 products; however, live bacteria overcome their stimulatory effects. Therefore, it is possible that OmpA interaction with gp96 on PMNs induces virulence factors in EC-K1 that are responsible for the prevention of oxidative burst. Our recent studies have shown that loops 1, 2 and 4 are important for interaction of OmpA with gp96 in HBMEC for EC-K1 invasion [50] . We also demonstrate that loop 2 interaction with PMNs is critical for survival of EC-K1 in vitro and for the establishment of meningitis [20] . In support of these studies, the data here demonstrate that loop 2 interaction of OmpA with gp96 controls the survival of the bacterium in PMNs. Lack of loop 2 interaction with gp96 enhanced the expression of CR3, which was subsequently used by the bacteria to enter PMNs. However, entry through CR3 resulted in complete elimination of bacteria from PMNs, indicating that loop 2–gp96 interaction activates signalling mechanisms for survival in PMNs. Similarly, EC-K1 interaction with macrophages suppresses the expression of CR3 during the onset of meningitis [35] . Of note, in macrophages, OmpA of EC-K1 interacts with Fc-gamma receptor I for entering the cells, although both Fc-gamma receptor I and gp96 expression increased on infection with EC-K1 [34] . In addition, we observed that depletion of PMNs at later stages of infection did not affect the outcome of EC-K1 meningitis. This suggests that EC-K1 finds a niche in PMNs for its multiplication during the initial stages and subsequently manipulates the function of macrophages to reach high-grade bacteremia. Therefore, PMNs and macrophages have an important role at different temporal stages of infection in the pathogenesis of EC-K1 meningitis. Taken together, these results suggest that EC-K1 exploits PMNs by interacting with gp96 via loop 2 of OmpA to suppress the anti-bactericidal activity of the cells. Therefore, blocking this initial interaction would be an attractive strategy for developing therapeutic avenues to preventing this deadly disease in neonates. Bacterial strains All strains used in this study were derived from a cerebrospinal fluid isolate of EC-K1 strain RS218 (serotype O18:K1:H7). E44 is spontaneous rifampin-resistant mutant of RS 218 strain (designated as OmpA + E. coli ) and E91 is a derivative of E44 that expresses no OmpA [10] . E91 (OmpA − E. coli ) was transformed with pUC19 containing the entire ompA gene and the pUC19 plasmid alone to obtain pOmpA + E. coli and pOmpA − E. coli , respectively. EC-K1 strains that lack S-fimbriae (Δsfa), type 1 fimbriae (ΔfimH), ibeA gene (ΔibeA), and CNF 1 (Δcnf) are described elsewhere [8] , [9] , [10] , [11] , [12] , [13] , [18] , [19] . All bacteria were grown in Luria broth with appropriate antibiotics, as necessary. Bacterial lysates were prepared by suspending EC-K1 strains in 0.5% Triton X-100 in PBS and sonicated briefly (30-s pulses) over a period of 3 min on ice. Cellular debris was removed by centrifugation followed by filtration through 0.2-μm pore-size filters. The absence of live bacteria was confirmed by plating the lysates on blood agar plates and incubation overnight at 37 °C. Isolation of human PMNs Heparinized venous blood was obtained from consented healthy volunteers following a protocol approved by the Children's Hospital Los Angeles Institutional Review Board. Dextran-sedimented PMNs were purified on a Ficoll–Hypaque gradient, as previously described [25] . PMNs were re-suspended at 1×10 7 cells per ml in Dulbecco's PBS (without calcium and magnesium; Mediatech) containing 0.1% dextrose and kept on ice until use. PMN preparations were >95% pure as determined by flow cytometry as well as cytospin preparations and morphological assessment by phase-contrast microscopy. PMNs were >99% viable as monitored by trypan blue exclusion and Annexin-V-PI staining. Determination of entry and intracellular bacteria in PMNs PMNs (1×10 6 cells ml −1 ) were washed three times in culture medium without antibiotics and varying concentrations of bacteria were added to the tubes. PMNs and bacteria were then incubated for 1 h at 37 °C. Gentamicin was added to PMN-bacteria co-culture tubes at a final concentration of 100 μg ml −1 and incubated for a further 60 min at 37 °C. PMN-bacteria co-cultures were washed 3 times in RPMI 1640 containing no antibiotics and reconstituted with antibiotic-free culture medium. Tubes were then assessed immediately for intracellular bacteria (time period 0) or placed again at 37 °C in culture medium containing 100 μg ml −1 gentamicin. To determine number of bacteria entered inside PMNs, PMN-bacteria co-cultures (described above) were washed twice and cells were lysed with 100 μl of 0.5% Triton X-100. The released intracellular bacteria were enumerated by plating 20 μl each of PMN-bacteria co-culture supernatant on blood agar plates. Counts in supernatant was subtracted from the initial count to calculate the number of bacteria entered inside PMNs [18] , [33] , [35] . Results are expressed as percentage of bacteria taken up by PMNs at respective sampling time intervals. Luminol-dependent chemiluminescence A total of 10 6 PMNs were incubated in Morse's defined medium [51] in the presence of 20 μM luminol (Sigma), at a final volume of 1 ml. For stimulation experiments, PMNs were incubated with live or heat-killed EC-K1 at a multiplicity of infection of 10 (cell to bacteria ratio, 1:10). Luminol-dependent chemiluminescence (LDCL) was measured in an LKB-Wallac 1250 luminometer (Perkin Elmer) every 5 min for 1 h at 37 °C, and the counts per second of LDCL were averaged per condition between triplicate tubes. Untreated and 10 ng ml −1 PMA-treated PMNs served as negative and positive controls, respectively, to determine ROS production. In some experiments, PMNs were pre-exposed to 10 mM diphenylidene iodonium hydrochloride (Sigma) for 10 min or XVA143 (10 μM) before the addition of bacteria for 1 h. XVA143, a β2 integrin allosteric antagonist (CR3 inhibitor), was generously provided by Dr N. Fotouhi (Roche) [52] . Experiments were repeated at least five times, using PMNs from a different donor for each triplicate. RT–PCR Total RNA from uninfected, E. coli -infected or PMA-treated human PMNs was isolated using RNA extraction kit (Qiagen) and then reverse transcribed using an RT–PCR kit (Qiagen). The primer sequences used were as follows: Rac1 (forward 5′-AGGAAGAGAAAATGCCTG-3′; reverse 5′-AGCAAAGCGTACAAA GGT-3′); Rac2 (forward 5′-TAGATGGGTCTGATCCTC-3′; reverse 5′-AGAAAAGACCATCAACGA-3′; gp91phox (forward 5′-ATGGGGAACTGGG CTGTGAAT-3′; reverse 5′- CCTC ATGGAAGAGACAAGTTAGAA-3′). Flow cytometry The levels of gp96, Rac1, Rac2 and gp91 phox in PMNs were determined by flow cytometry. The cells were fixed and permeabilized in cytofix and cytoperm buffer (BD Biosciences) followed by incubation with IgGblocking buffer-to-mask nonspecific binding sites. After incubation, cells were incubated with gp96, Rac1 (Abcam), Rac2 or gp91phox (Santa Cruz biotechnology) antibody. The cells were then washed and incubated with secondary antibody conjugated to Alexa Fluor 488 antibody (Invitrogen). For extracellular staining of gp96, cells were fixed in cytofix, washed, incubated with IgG-blocking buffer followed by incubation with primary and secondary antibodies. gp96 antibody was generated in our laboratory as described earlier [10] . The cells were then analysed by flow cytometry using FACS Calibur Cell Quest Pro software (BD Biosciences) and at least 10,000 events were gated. siRNA transfection PMNs were transfected with CR3 siRNA (oligo identification number HSS179976) or gp96 siRNA (oligo identification numbers HSS110955 (gp96-siRNA-1), HSS110953 (gp96- siRNA-2) and HSS186409 (gp96-siRNA-3), Invitrogen) using Lipofectamine 2000 plus (Invitrogen) according to the manufacturer's instructions. Briefly, 20 pmols of CR3 or gp96 siRNA in 100 μl of Lipofectamine 2000 plus was added to PMNs (5×10 5 ) suspended in Opti-MEM I reduced-serum medium (Invitrogen) having no antibiotics and incubated at 37 °C for 6 h. After incubation, the medium was replaced with RPMI 1640 containing L-Glutamine, sodium pyruvate, nonessential amino acids, 1% penicillin/streptomycin, and 10% fetal calf serum. Cells were collected 24 h after transfection and CR3 or gp96 knockdown was determined by flow cytometry. The viability of the cells was assessed by trypan blue exclusion and Annexin-V-PI staining that revealed >90% viability of the transfected cells. Newborn mouse model of meningitis The animal studies were approved by the Institutional Animal Care and Use Committee of the Saban Research Institute at Children's Hospital Los Angeles and followed National Institutes of Health guidelines for the performance of animal experiments. Breeding pairs of C57BL/6 wild-type mice were obtained from Jackson Laboratories. Three-day-old mouse pups were randomly divided into various groups and infected intranasally with different doses of bacteria or pyrogen free saline [33] , [35] , [53] . Blood was collected from the tail or facial vein at different time periods of post-infection; dilutions were made; and plated on rifampicin LB agar plates. CSF samples were collected aseptically by cisternal puncture under anesthesia and directly inoculated into broth containing appropriate antibiotics. Bacterial counts in blood and brain tissue homogenates were determined by plating tenfold serial dilutions on rifampicin LB agar plates. Growth of EC-K1 in rifampicin-containing LB broth from CSF samples was considered positive for meningitis. PMNs were depleted in mice by the administration of mAb RB6-8C5 as described in earlier studies [32] , [54] . Mice were given a total of 4 doses of RB6, 2 doses at 12 h interval (100 μg) on day 1 and similar doses at day 2 and infected with EC-K1 on day 3. Control group received similar doses of isotype-matched antibody. PMNs were also depleted in EC-K1-infected mice 24 h post-infection by injecting 2 doses of RB6-8C5 antibody 6 h apart. Similar doses of isotype-matched antibody were injected in control mice. The depletion of PMNs was confirmed by flow cytometry using anti-Gr1 antibody. Suppression of gp96 expression in newborn mice gp96 expression was suppressed in neonatal mice by siRNA to gp96 and Invivofectamine, as described earlier [35] , [53] . Briefly, newborn mice were given four doses of gp96 siRNA (10 nmol; oligo identification number MSS205545, Invitrogen) intraperitoneally; two doses before infection on day 1 and day 2, one dose immediately after administration of bacteria on day 3, and final dose at 24 h after infection on day 4. The suppression of gp96 in splenic PMNs on day 3 and day 4 was confirmed by flow cytometry and RT–PCR. Determination of BBB leakage The quantitative evaluation of BBB permeability was done by detection of extravasated Evans blue dye [33] , [55] . Briefly, mice were injected intraperitoneally with 2% Evans blue dye in saline and, after 4 h, animals were deeply anaesthetized with Nembutal and transcardially perfused until colourless perfusion fluid was obtained from the right atrium. After decapitation, brain tissue was removed, weighed, homogenized and centrifuged. The protein concentration was then determined in the tissue supernatants. Evans blue intensity was determined by a microplate reader at 550 nm. Results were expressed in micrograms of Evans blue dye per mg protein. Statistical analysis Statistical significance was determined by a paired, two-tailed Student's t -test, ANOVA and Fisher's exact test. Values of P <0.05 were considered to be statistically significant. How to cite this article: Mittal, R. et al . gp96 expression in neutrophils is critical for the onset of Escherichia coli K1 (RS218) meningitis. Nat. Commun. 2:552 doi: 10.1038/ncomms1554 (2011).